Programmable spin-state switching in a mixed-valence spin-crossover iron grid Photo-switchable systems, such as discrete spin-crossover complexes and bulk iron–cobalt Prussian blue analogues, exhibit, at a given temperature, a bistability between low- and high-spin states, allowing the storage of binary data. Grouping different bistable chromophores in a molecular framework was postulated to generate a complex that could be site-selectively excited to access multiple electronic states under identical conditions. Here we report the synthesis and the thermal and light-induced phase transitions of a tetranuclear iron(II) grid-like complex and its two-electron oxidized equivalent. The heterovalent grid is thermally inactive but the spin states of its constituent metal ions are selectively switched using different laser stimuli, allowing the molecule to exist in three discrete phases. Site-selective photo-excitation, herein enabling one molecule to process ternary data, may have major ramifications in the development of future molecular memory storage technologies. Bistable materials, which have two thermodynamically stable phases at a given temperature, have switchable electronic states that can be manipulated through the application of external stimuli and may have major applications in future technologies as quantum logic operators or components in memory storage devices [1] , [2] , [3] . The (SCO) phenomenon, by which transition metal ions can exhibit magnetic bistability, has been reported in a wide range of systems, from mononuclear complexes to infinite coordination polymers [4] , [5] . Complexes of transition metal ions with d 4 to d 7 electronic configurations may show reversible SCO between their high-spin (HS) and low-spin (LS) states when stimulated by temperature, light, pressure or guest absorption/desorption [6] , [7] . Their simple synthesis and functionality have made them excellent candidates as molecular switches or sensors [8] . Iron(II) complexes are the most commonly reported thermal SCO materials [9] , but there are various examples based on other metal ions [10] , [11] , [12] , [13] , [14] . Iron(II) complexes also exhibit a light-induced LS→HS state transition (LIESST: light-induced exited spin-state trapping) [15] , but usually only at low temperatures. The meta-stable HS state is generated by excitation of the d – d or metal-to-ligand charge transfer (MLCT) absorption band, changing the spin state of the iron(II) ion from S LS =0 to S HS =2. The associated elongation (~0.2 Å) of the coordination bond lengths energetically disfavours thermal relaxation back to the LS state at low temperature, allowing the light-induced meta-stable state to be trapped [16] , [17] . LIESST has also been seen in iron(III) SCO complexes, usually through excitation of the ligand-to-metal charge transfer (LMCT) band, but the shorter associated average (LS to HS) bond elongation (~0.1 Å) can make the meta-stable HS state more difficult to trap [18] . Systems incorporating multiple bistable building units may display more than two stable phases when stimulated by heat or light, and have the potential to act as multi-responsive, multi-faceted [19] or selective switches in nano-scale devices [20] . Approaches to the generation of multi-bistable systems include the crystallization of mononuclear SCO complexes in asymmetric packing environments [21] , the co-crystallization of different bistable molecules [22] and the linkage of two or more bistable building blocks in a molecular system, in which the stabilization of an intermediate state depends on the degree to which neighbouring chromophores are electronically coupled [23] . Cooperative SCO behaviour, mediated by the steric and electronic stress applied to neighbouring metal centres by multidentate or bridging ligands, has been reported in dinuclear complexes [23] , tetranuclear squares [24] , [25] and grid-like complexes [26] , [27] , [28] . Indeed, the study of grid-type clusters is of particular interest, as their tunable electronic states [29] , [30] have seen them proposed as quantum cellular automata; molecular binary logic devices that function through coulombic interactions between metal centres on neighbouring cells [31] . Intramolecular electronic cooperativity in {Fe II 4 } grids (consisting of four equivalent chromophores) has been shown to lead to multi-step thermal SCO, as geometric and electronic changes associated with each spin transition have knock-on effects on the electronic states of the neighbouring metal ions [27] . Step-wise thermal conversion does not, however, guarantee that multiple discrete phases can be accessed photochemically. To address this, our strategy is to develop a molecule containing different SCO-active chromophores, which will allow the cluster to exist in three discrete light-accessible states at low temperatures, that is, below ~50 K ( Fig. 1 ). Aromatic imidazolate ligands are used to bridge Fe II and Fe III SCO chromophores in a grid-type architecture and, as anticipated, the heterovalent ions are selectively excited by different laser stimuli, thus creating, to the best of our knowledge, the first example of site-selective spin-state switching. 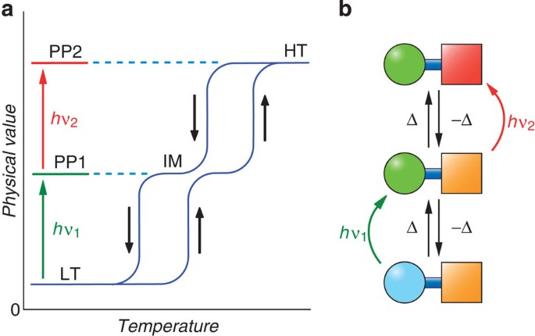Figure 1: Multi-bistability. Representative plot (a) and scheme (b) of the adopted approach to the synthesis of selectively photo-excitable molecules, in which different SCO-active chromophores are incorporated into the same structure. HT, IM and LT are the high, intermediate and low temperature (thermally accessible) phases, respectively, and PP1 and PP2 are the first and second photo-induced phases, respectively. The thermal multi-bistability is represented by the blue trace, which undergoes two hysteretic transitions, from HT to LT via an IM phase. The corresponding photochemical phases, PP1 and PP2, accessed by irradiation at wavelengthshν1andhν2, are represented by green and red traces, respectively. The scheme (b) illustrates the possible thermal (Δ) phase transitions and how the chromophores are selectively excited by the different wavelengths of light (hν1andhν2). Figure 1: Multi-bistability. Representative plot ( a ) and scheme ( b ) of the adopted approach to the synthesis of selectively photo-excitable molecules, in which different SCO-active chromophores are incorporated into the same structure. HT, IM and LT are the high, intermediate and low temperature (thermally accessible) phases, respectively, and PP1 and PP2 are the first and second photo-induced phases, respectively. The thermal multi-bistability is represented by the blue trace, which undergoes two hysteretic transitions, from HT to LT via an IM phase. The corresponding photochemical phases, PP1 and PP2, accessed by irradiation at wavelengths h ν 1 and h ν 2 , are represented by green and red traces, respectively. The scheme ( b ) illustrates the possible thermal (Δ) phase transitions and how the chromophores are selectively excited by the different wavelengths of light ( h ν 1 and h ν 2 ). Full size image Syntheses and structures The bridging ligand 2-phenyl-4,5-bis{6-(3,5-dimethyl-1H-pyrazol-1-yl)pyrid-2-yl}-1H-imidazole ( HL ) was synthesized from the condensation of 2,6-dibromopyridine and 3,5-dimethyl-1H-pyrazole following a five-step pathway ( Fig. 2 and Methods). The reaction of Fe(BF 4 ) 2 ·6H 2 O and HL in acetonitrile yielded a red solution, from which orange rhombic crystals suitable for the single-crystal X-ray structural determination of [Fe II 4 (L) 4 ](BF 4 ) 4 ·2CH 3 CN ( [Fe II 4 ] ) were obtained by diethyl ether diffusion ( Fig. 3 ). Cyclic voltammetry measurements of [Fe II 4 ] were carried out in acetonitrile at 293 K ( Fig. 4 , inset), and showed four quasi-reversible redox waves at E 1/2 =+0.52 V, +0.61 V, +0.90 V and +1.00 V (versus saturated calomel electrode (SCE)) corresponding to the one-electron oxidation of the four iron centres. The comproportionation constant of the two-electron oxidized complex {Fe III 2 Fe II 2 } 6+ was 9.8 × 10 4 (ref. 32 ), suggesting that the mixed-valence species was relatively stable in acetonitrile. [Fe II 4 ] was, therefore, chemically oxidized using excess AgBF 4 in nitromethane to yield, after filtration and slow diffusion of diethyl ether, dark red crystals of [Fe III 2 Fe II 2 (L) 4 ](BF 4 ) 6 ·6CH 3 NO 2 ·(C 2 H 5 ) 2 O·4H 2 O ([Fe III 2 Fe II 2 ]). 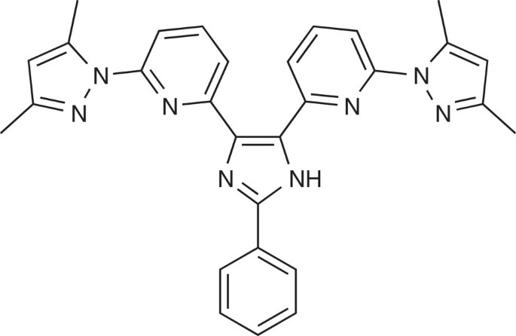Figure 2: Structure of ligand HL. The central imidazole moiety bridges two discrete tridentate-binding sites. Figure 2: Structure of ligand HL. The central imidazole moiety bridges two discrete tridentate-binding sites. 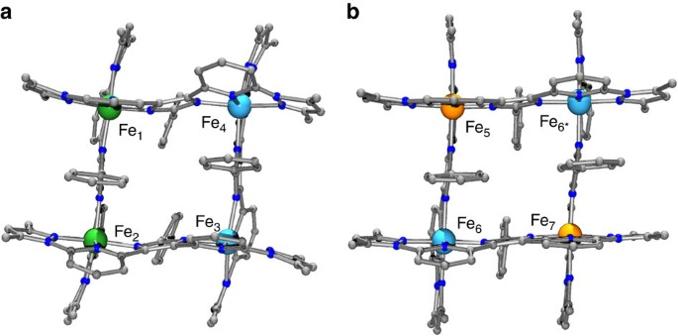Figure 3: Crystal structures of[FeII4]and [FeIII2FeII2]. (a)[FeII4](position A) and (b) [FeIII2FeII2] at 100 K. HS-FeIIcentres are shown in green; LS FeII, sky-blue; LS-FeIII, orange; C, grey and N, blue. For clarity, counteranions, hydrogen atoms and solvent molecules have been omitted. Full size image Figure 3: Crystal structures of [Fe II 4 ] and [Fe III 2 Fe II 2 ]. ( a ) [Fe II 4 ] (position A) and ( b ) [Fe III 2 Fe II 2 ] at 100 K. HS-Fe II centres are shown in green; LS Fe II , sky-blue; LS-Fe III , orange; C, grey and N, blue. For clarity, counteranions, hydrogen atoms and solvent molecules have been omitted. 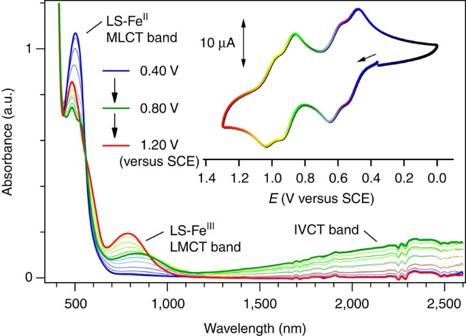Figure 4: Controlled potential absorption spectra of[FeII4]. The absorption spectra show three key processes on increasing the applied potential from 0.5 to 1.2 V: a decrease in LS-FeIIMLCT band (501 nm) intensity, an increase in LS-FeIIILMCT band (864 nm) intensity, and the appearance and subsequent disappearance of an IVCT band (>2,000 nm). Inset: CV data of[FeII4]. Full size image Figure 4: Controlled potential absorption spectra of [Fe II 4 ] . The absorption spectra show three key processes on increasing the applied potential from 0.5 to 1.2 V: a decrease in LS-Fe II MLCT band (501 nm) intensity, an increase in LS-Fe III LMCT band (864 nm) intensity, and the appearance and subsequent disappearance of an IVCT band (>2,000 nm). Inset: CV data of [Fe II 4 ] . Full size image The crystallographically determined structures of [Fe II 4 ] and [Fe III 2 Fe II 2 ] are shown in Fig. 3 . [Fe II 4 ] crystallized in the P space group and temperature-dependent structural data were collected at 18, 100 and 190 K (in heating mode) and at 293 K. [Fe II 4 ] has a tetranuclear grid-like core, consisting of four crystallographically independent iron ions and ligands. The ligands adopt bis-tridentate coordination modes, bridging the iron ions through their central imidazolate moieties, ensuring that all four iron ions are coordinated by two tridentate-binding sites, resulting in N 6 coordination environments. Structural data collected at both 18 K ( Supplementary Fig. 1 ; Supplementary Table 1 ) and 100 K ( Supplementary Fig. 2 ; Supplementary Table 2 ) allowed the characterization of the cluster in two partially occupied, overlaid configurations (A and B), leading to relatively low precision on the observed bond distances. Despite this, the bond lengths and angular distortion parameters (Σ) allowed us to suggest that Fe1A and Fe2A were HS and Fe3A and Fe4A were LS ions, while Fe1B and Fe4B were HS and Fe2B and Fe3B were in the LS state; a ratio confirmed by low temperature magnetic susceptibility and Mössbauer data ( Fig. 5 , Supplementary Fig. 3 ; Supplementary Table 3 ). In both configurations, the grid had a cis -2HS-2LS configuration, abbreviated as [(HS-Fe II ) 2 (LS-Fe II ) 2 ], similar to that described in the first crystallographically determined 2HS-2LS iron grid and the subsequent theoretical studies thereupon [33] , [34] , although more recently a trans -2HS-2LS grid has also been reported [35] . Increasing the measurement temperature from 100 K to 190 K caused the c axis to double in length, and the unit cell to contain two crystallographically independent sites, both of which were occupied by two overlaid cluster configurations (see Supplementary Fig. 4 ; Supplementary Table 4 ) [36] , [37] , [38] . Once again, the large number of atoms led to relatively low precision on the bond distances. At site 1, in both configurations A and B, the bond lengths and angles suggested that ion Fe3A/B was in the LS state, while all other ions were in the HS state. At the second site, molecule C contained two LS ions at positions Fe2C and Fe4C, while all ions in molecule D were in the HS state. Overall, the intermediate (IM) phase can be represented by the average formula [(HS-Fe II ) 3 (LS-Fe II )], a ratio confirmed by magnetic susceptibility and Mössbauer data ( Fig. 5 , Supplementary Fig. 3 ; Supplementary Table 3 ). Increasing the measurement temperature to 293 K completed the transition to the [(HS-Fe II ) 4 ] HT phase (HS-Fe II -N av =2.17(1) Å). Temperature-dependent crystallographic analysis showed that [Fe II 4 ] displayed two-step intramolecular SCO behaviour while retaining single crystallinity, allowing us to follow the spin-state changes on each metal site as a function of temperature. 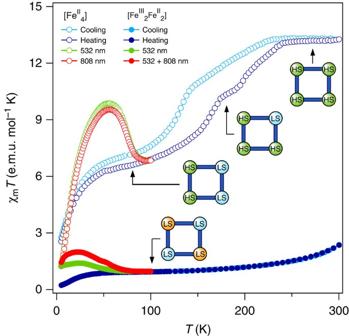Figure 5: Magnetic susceptibility measurements. The thermal and light-induced magnetic susceptibility data collected for[FeII4](empty markers; dark blue, heating mode; light blue, cooling mode; green, 532 nm laser; red, 808 nm laser) and [FeIII2FeII2] (filled markers; blue, heating mode; light blue, cooling mode; green, 532 nm laser; red, 532 then 808 nm lasers). [FeIII2FeII2] showed very little thermal phase transition, but irradiation with the different lasers had contrasting effects on the low temperature χmTvalues. Figure 5: Magnetic susceptibility measurements. The thermal and light-induced magnetic susceptibility data collected for [Fe II 4 ] (empty markers; dark blue, heating mode; light blue, cooling mode; green, 532 nm laser; red, 808 nm laser) and [Fe III 2 Fe II 2 ] (filled markers; blue, heating mode; light blue, cooling mode; green, 532 nm laser; red, 532 then 808 nm lasers). [Fe III 2 Fe II 2 ] showed very little thermal phase transition, but irradiation with the different lasers had contrasting effects on the low temperature χ m T values. Full size image [Fe III 2 Fe II 2 ] crystallized in the monoclinic space group C 2/ c at 100 K ( Fig. 3 ). The oxidation and spin states of the iron ions in [Fe III 2 Fe II 2 ] were confirmed by charge balance, magnetic susceptibility measurements and Mössbauer spectra. The grid was diagonally bisected by a C 2 axis, resulting in three crystallographically independent iron ions, suggesting that homovalent ions were likely to be found on opposite corners. The Mössbauer spectrum of [Fe III 2 Fe II 2 ] collected at 100 K confirmed that LS-Fe III and LS-Fe II ions existed in a 1/1 ratio in the grid, and the observation of two LS-Fe III doublets and one LS-Fe II doublet suggested that the Fe III ions were located on the crystallographically inequivalent Fe5 and Fe7 positions (see Supplementary Fig. 5 ; Supplementary Table 5 ). The average coordination bond lengths around the iron ions at 100 K were Fe5=1.948(3) Å, Fe6=1.957(3) Å and Fe7=1.940(3) Å, respectively, suggesting that all iron ions were in the low-spin state at 100 K. Increasing the data collection temperature to 250 K caused structural disorder around the Fe7 centre, indicative of incomplete single-site Fe III spin transition, an observation in line with the Mössbauer spectra, in which a low-intensity HS-Fe III doublet progressively appeared as temperature was increased (see Supplementary Fig. 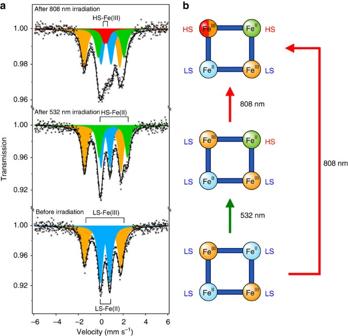Figure 6:57Fe Mössbauer spectroscopy. (a) The light irradiation-dependent57Fe Mössbauer spectra of [FeIII2FeII2] at 5 K. (b) The Mössbauer spectra confirm that irradiation with 532 nm (green) laser results in FeII-specific LIESST, while subsequent irradiation with 808 nm (red) laser light causes spin transitions to occur on the FeIIIions. 6 ; Supplementary Table 6 ). Controlled potential absorption spectra Full understanding of the relevant electronic transition energies within the molecules was key if selective LIESST was to be observed. The room temperature solution-state absorption spectra of [Fe II 4 ] and [Fe III 2 Fe II 2 ] were comparable with those obtained from powdered samples at 100 K, suggesting that the complexes were in their LT phases in solution (see Supplementary Figs 7 and 8 ). Controlled potential Ultraviolet–visual measurements were conducted on a solution of [Fe II 4 ] in acetonitrile to track the absorption bands associated with all accessible redox states ( Fig. 4 ). Initial oxidation from {Fe II 4 } 4+ to {Fe III 2 Fe II 2 } 6+ caused the LS-Fe II MLCT band ( λ max =501 nm) to weaken, while new absorption bands appeared at 864 nm and 2,462 nm. Full oxidation to a {Fe III 4 } 8+ species caused the band at 2,462 nm to disappear, while that at 864 nm increased in intensity underwent a blue-shift, indicating the absorption at 2,462 nm to be an intervalence charge transfer (IVCT) band between heterovalent iron ions, and the band at 864 nm to be the LS-Fe III LMCT band [39] . Absorption spectra were collected from single crystals of [Fe II 4 ] to observe the low-energy edge of the LS-Fe II MLCT band at high resolution, and showed it to extend to around 850 nm (see Supplementary Fig. 9 ). The observation of the discrete MLCT (501 nm) and LMCT (864 nm) bands in the spectra corresponding to the {Fe III 2 Fe II 2 } 6+ species suggested that site-selective LIESST would be possible in [Fe III 2 Fe II 2 ]. Temperature-dependent magnetic susceptibility Magnetic susceptibility measurements were carried out on [Fe II 4 ] and [Fe III 2 Fe II 2 ] in heating ( ↑ ) and cooling ( ↓ ) modes ( Fig. 5 ). [Fe II 4 ] exhibited multi-step thermal SCO, in agreement with the temperature-dependent structural data, from [(HS-Fe II ) 4 ] at room temperature, via a [(HS-Fe II ) 3 (LS-Fe II )] intermediate plateau, to [(HS-Fe II ) 2 (LS-Fe II ) 2 ] at around 100 K. For [Fe III 2 Fe II 2 ], the χ m T value at 100 K was 0.942 e.m.u. mol −1 K, closely matching the predicted value of 1.00 ( g =2.31) for two uncorrelated LS-Fe III ions ( S =1/2) and two LS-Fe II ions ( S =0). With heating, the χ m T value increased gradually, reaching 2.36 e.m.u. mol −1 K at 300 K. Further heating led to some sample degradation, so all measurements were carried out below 300 K. The susceptibility data suggest that thermal SCO occurred gradually above 200 K, in agreement with the structural and Mössbauer analyses [40] . The decrease in χ m T values at low temperature indicates that antiferromagnetic interactions were operative between the LS-Fe III ions, and fitting the data collected in heating mode up to 100 K gave a J value of −2.47(9) cm −1 and a g value of 2.31; the small J value, which may include both intra- and inter-molecular interactions, supports the assignment of trivalent ions on opposite corners of the grid ( Supplementary Fig. 10 ). The LS-Fe II ions in [Fe III 2 Fe II 2 ] show greater thermal stability than those in [Fe II 4 ] , probably attributable to the more pronounced distortion of the Fe II coordination environments in [Fe II 4 ] (see Supplementary Table 7 ) [41] , [42] . Selective photoswitching The combination of heterovalent iron chromophores within a SCO complex suggested that, for the first time, site-specific LIESST would be accessible. To investigate the wavelength-dependent photo-response of [Fe II 4 ] and [Fe III 2 Fe II 2 ], irradiation experiments were conducted inside the SQUID magnetometer. For the LIESST phenomenon to be observed, specific electronic absorption bands should be excited; usually d – d or MLCT for Fe II and LMCT for Fe III . Ultraviolet–visible–near infrared measurements showed [Fe II 4 ] to have a broad MLCT band centred at λ max =501 nm and spreading to ca. 850 nm, while [Fe III 2 Fe II 2 ] had a separate LMCT band at 864 nm originating from its LS-Fe III moieties (see Supplementary Figs 7–9 ). These observations formed the basis for our site-selective LIESST excitation experiments. Irradiation of a microcrystalline sample of [Fe II 4 ] at 532 nm (10 mW cm −2 ) at 5 K caused the initial χ m T value to decrease ( Fig. 5 ). As the sample was heated to 56 K, the χ m T value increased rapidly to a maximum of 9.87 e.m.u. mol −1 K, indicating the occurrence of the LIESST effect due to excitation of the LS-Fe II MLCT band. The photo-induced state then thermally relaxed to the initial phase on further temperature increase. When 808 nm laser irradiation (10 mW cm −2 ) was used, very similar behaviour was observed, with a χ m T maximum of 9.54 e.m.u. mol −1 K at 56 K. This behaviour is attributable to the excitation of the low-energy tail of the broad LS-Fe II MLCT band discussed above. For [Fe III 2 Fe II 2 ], a green light-induced excited state was accessed by irradiation with a 532 nm laser (10 mW cm −2 ) at 5 K, which led to an increase in the χ m T values, reaching a saturation value of 1.24 e.m.u. mol −1 K after 4 h (see Supplementary Fig. 11 ). When the sample was then irradiated with red light (10 mW cm −2 ) at 5 K, the χ m T value increased to a second saturation level of 1.46 e.m.u. mol −1 K indicative of a second green+red light-induced excited state (g+rES). Subsequent temperature increases were mirrored by rises in the χ m T values of both the green light-induced excited state and g+rES, indicative of antiferromagnetic coupling, reaching maxima at 22 K of 1.40 and 1.99 e.m.u. mol −1 K, respectively, before thermally relaxing to the LS phase. Both species had entirely reverted to the ground state by 100 K. When [Fe III 2 Fe II 2 ] was excited by only red light, the susceptibility reached saturation at 1.45 e.m.u. mol −1 K after 6 h; very close to the value obtained for the g+rES. It should be noted that the relatively low χ m T values reached on irradiation are likely to be due in part to the existence of strong intramolecular antiferromagnetic coupling, originating from the charge transfer interactions, between the heterovalent metal centres. [Fe III 2 Fe II 2 ] can be considered a thermally inactive photo-switchable material, an unusual observation in SCO materials research [43] . Due to the low relaxation temperature and the existence of the intramolecular antiferromagnetic interactions at low temperature, the spin states of the excited species could not be elucidated by susceptibility data alone. Light irradiation experiments were carried out on single crystals of [Fe II 4 ] and [Fe III 2 Fe II 2 ]. Irradiation at 532 and 808 nm to a single crystal of [Fe II 4 ] caused the bond distances to increase to lengths similar to those seen at 293 K, characteristic of full [(HS-Fe II ) 2 (LS-Fe II ) 2 ]→[(HS-Fe II ) 4 ] transition (see Supplementary Table 8 ). No structural change was observed, however, on radiation of [Fe III 2 Fe II 2 ] crystals, probably as a result of their dark colour and impenetrability to light. To investigate the electronic characteristics of the light-induced excited states with maximum sensitivity, 57 Fe (95.5%)-enriched samples of [Fe II 4 ] and [Fe III 2 Fe II 2 ] were prepared. Mössbauer measurements conducted at 5 K on [Fe II 4 ] (LS-Fe II /HS-Fe II =1/1) indicated that irradiation at 532 nm and 808 nm resulted in similar LS-Fe II /HS-Fe II ratios of 0.18/0.82 and 0.17/0.83, respectively (see Supplementary Fig. 12 ; Supplementary Table 9 ). It should be noted that the deviation of these values from a 0/1 ratio might be due to the difficulties associated with ensuring complete sample exposure inside the Mössbauer spectrometer. The Mössbauer spectrum of [Fe III 2 Fe II 2 ] collected in the absence of light at 5 K showed two doublet peaks corresponding to LS-Fe II and LS-Fe III species, with a peak-intensity ratio of LS-Fe III /LS-Fe II =0.45/0.55 ( Fig. 6 ; Supplementary Table 10 ). After 532 nm laser irradiation at 5 K, however, the LS-Fe II absorption decreased, and a new doublet appeared corresponding to HS-Fe II . The peak-intensity ratio of LS-Fe III /HS-Fe III /LS-Fe II /HS-Fe II =0.42/0.00/0.31/0.27 confirmed that Fe II -specific LIESST had occurred after exposure to green light. The sample was then irradiated with 808 nm laser light at 5 K causing the intensity of the LS-Fe III doublet peak to decrease, and a new doublet peak to emerge with a small quadrupole-splitting parameter corresponding to HS-Fe III . The peak-intensity ratio of LS-Fe III /HS-Fe III /LS-Fe II /HS-Fe II =0.32/0.13/0.30/0.25, confirmed that red light stimulated LIESST of the Fe III ions. The Mössbauer data indicated that 532 and 808 nm lasers selectively induced LS-Fe II to HS-Fe II and LS-Fe III to HS-Fe III conversions, respectively, allowing a remarkable tetranuclear cluster to be generated in which iron ions are present in four different electronic states. It should be noted that when the sample was irradiated with only red laser light, the same result was obtained as when green+red lasers were used; this is explained by the overlapping absorption bands of the LS-Fe III LMCT and LS-Fe II MLCT transitions. Figure 6: 57 Fe Mössbauer spectroscopy. ( a ) The light irradiation-dependent 57 Fe Mössbauer spectra of [Fe III 2 Fe II 2 ] at 5 K. ( b ) The Mössbauer spectra confirm that irradiation with 532 nm (green) laser results in Fe II -specific LIESST, while subsequent irradiation with 808 nm (red) laser light causes spin transitions to occur on the Fe III ions. Full size image Homovalent ( [Fe II 4 ] ) and heterovalent ([Fe III 2 Fe II 2 ]) grids were synthesized and found to display LIESST at low temperatures. Although [Fe II 4 ] showed hysteretic multi-step thermal SCO behaviour, [Fe III 2 Fe II 2 ] showed little thermal SCO up to 300 K. Irradiation of [Fe III 2 Fe II 2 ] at low temperatures with green and red lasers led to Fe II - and Fe III -specific LIESST phenomena, respectively; this being the first observation of site-selective spin-state switching. The phenomenon of site-selective spin-state transition allows the electronic state of a molecule to be photochemically programmed between multiple levels. Molecules displaying such extraordinary multistability have great potential in future technologies as nano-scale logic devices, and the extension of such clusters into patterned arrays raises the possibility of light-programmable molecular memory with vast data storage density. X-ray crystallography A single crystal was removed from the mother liquor, mounted on a glass rod and intensity data were collected at 293 K, 190 K, 100 K, 18 K (dark, after irradiation 532 nm, and 808 nm laser) for the divalent species, and at 250 K, and 100 K for the mixed-valence compound, using a Bruker SMART APEX II CCD system with Mo-Kα radiation ( λ =0.71073 Å, 50 kV, 24 mA). See Supplementary Table 11 for all parameters. The structures were solved by direct methods and refined by full-matrix least-square techniques on F 2 using SHELXTL. All data sets were treated with the SQUEEZE program from the PLATON suite to remove highly disordered solvent molecules from the calculations. In all [Fe II 4 ] structures, electron density accounting for two acetonitrile molecules per formula unit was removed, while electron densities equivalent to two nitromethane and four water molecules, and four water molecules, were removed from the data sets of [Fe III 2 Fe II 2 ] at 250 K and 100 K, respectively. See Supplementary Note 1 ; Supplementary Data 1 . Magnetic measurements Susceptibility data were collected under an applied magnetic field of 500 Oe using a Quantum Design MPMS-5S SQUID magnetometer. The temperature dependence was measured at 3.0 K increments in settle mode. The scan rate of the temperature was fixed to 10.0 K min −1 above 10 K, and at 2.0 K min −1 below 10 K, and each measurement was performed 30 s after the temperature had stabilized. Magnetic data were corrected for the diamagnetism of the sample holder and of the sample using Pascal’s constants. In the light irradiation experiments, a small amount of sample was used to maximize the light conversion ratio. The sample was irradiated at 5 K by a DPSS laser (532 nm with 10 mW cm −2 , Opto Tech 532.200.KE.01 and 808 nm with 10 mW cm −2 , Intelite I808-120G-CAP) through an optical fibre (Newport F-MBD; 3 m length, 1.0 mm core size, 1.4 mm diameter). During irradiation, the magnetic moment was recorded at regular time intervals until saturation, after which point the light irradiation was stopped. The temperature dependence of magnetic susceptibility after light irradiation was measured using an applied magnetic field of 500 Oe and a scan rate of 0.1 K min −1 in sweep mode. Mössbauer spectra Mössbauer experiments were carried out using a 57 Co/Rh source in a constant-acceleration transmission spectrometer (Topologic Systems) equipped with an Iwatani HE05/CW404 cryostat. The spectrometer was calibrated using standard α -Fe foil. All samples for Mössbauer experiments were obtained using 57 Fe-enriched starting materials (95.5%). In the light irradiation experiments, the sample was irradiated at 5 K by a DPSS laser. Single-crystal absorption spectroscopy A specially designed spectrometer with a 25-cm-grating monochromator (JASCO M25-GT) and an optical microscope was used. A 150-W tungsten–halogen lamp and a 250-W xenon lamp were employed as the light sources, and Si and Ge photodiodes were used with a photomultiplier as the detectors. The light sources and detectors were selected depending on the measured energy range. Samples were cooled in a conduction-type cryostat. Cyclic voltammetry Cyclic voltammetry measurements were carried out in a standard one-compartment cell under a nitrogen atmosphere at 20 °C equipped with a platinum wire counter electrode, an SCE reference electrode, and a glassy carbon working electrode using a BAS 620A electrochemical analyzer. The measurements were performed in acetonitrile with 0.1 M tetra- n -butylammonium hexaflourophosphate ( n -Bu 4 NPF 6 ) as the supporting electrolyte at a scan rate of 50 mV s −1 . Ultraviolet–visible–near infrared spectroscopy Ultraviolet–visible–near infrared absorption spectra were recorded on Shimadzu UV-3150 spectrometer. The variable temperature dependence of ultraviolet–visible–near infrared spectra was measured on KBr pellet samples using the Shimadzu UV-3150 spectrometer equipped with a Unisoku USP-203-A cryostat. Controlled potential spectroscopy Controlled potential spectroscopy experiments were done in a 0.5-mm path length quartz cell under a nitrogen atmosphere. A BAS 620A electrochemical analyzer was used as a potentiostat. Electrochemical experiments were performed in a three-electrode cell containing a platinum-mesh working electrode, a platinum wire counter electrode and the SCE reference electrode. Controlled potential spectra were recorded with a Shimadzu UV-3150 spectrometer. The measurements were performed in acetonitrile with 0.1 M tetra- n -butylammonium hexaflourophosphate as the supporting electrolyte. NMR measurements 1 H NMR and 13 C NMR spectra were measured on a Bruker AVANCE400 spectrometer at room temperature. Chemical shifts in the NMR were reported in ppm ( δ ), relative to the internal standard of tetramethylsilane. The signals observed were described as s (singlet), d (doublet), t (triplet), m (multiplets). The number of protons ( n ) for a given resonance is indicated as n H. Coupling constants are reported as J in Hz. Elemental analysis Elemental analyses were performed using a Perkin Elmer 2400 element analyzer. General synthesis All reagents were obtained from commercial suppliers and were used without further purification except when noted, or additionally distilled (diglyme (bis(2-methoxyethyl)ether) over calcium hydride and diethyl ether over sodium/benzophenone) as required. For a scheme of the synthesis of HL see Supplementary Fig. 13 . Preparation of 2-bromo-6-(3,5-dimethyl-1H-pyrazol-1-yl)pyridine (1) A solution of 3,5-dimethyl-1H-pyrazol (8.00 g, 83.2 mmol) in anhydrous diglyme (200 cm 3 ) was stirred at 70 °C with sodium (1.80 g, 79.0 mmol) until the metal dissolved. To this solution was added 2,6-dibromopyridine (20.0 g, 84.4 mmol) in one portion. The resulting mixture was stirred at 60 °C for 42 h. The solvent was removed in vacuo , and water (200 cm 3 ) was added. A crude white precipitate was collected by filtration and dried. The solid was purified by column chromatography on silica gel (eluting with dichloromethane) to give 1 (12.2 g, 48.3 mmol, 61% yield) as a crystalline white solid [44] : 1 H NMR (CDCl 3 ) δ 7.84 (d, 1H, J =8.0 Hz), 7.60 (dd, 1H, J =7.8 Hz), 7.29 (d, 1H, J =7.2 Hz), 5.99 (s, 1H), 2.65 (s, 3H), 2.28 (s, 3H). Anal. (calc.) for C 10 H 10 N 3 Br ( 1 ): C, 47.81 (47.64); H, 4.07 (4.00); N, 16.69 (16.67)%. Preparation of 6-(3,5-dimethyl-1H-pyrazol-1-yl)-2-pyridinecarboxylaldehyde (2) 1 (10.1 g, 40.0 mmol) was dissolved in anhydrous diethyl ether (150 cm 3 ) under a nitrogen atmosphere. The solvent was cooled down to −78 °C and n -buthyl lithium (2.6 M in hexane) (15.4 cm 3 , 40.0 mmol) was added slowly, keeping the temperature under −60 °C. After stirring for 1 h at −78 °C, anhydrous N,N-dimethylformamide (6.74 cm 3 , 87.1 mmol) was added, ensuring that the reaction temperature did not exceed −70 °C. The mixture was stirred for one further hour at −78 °C, before the reaction was quenched by the addition of 6 M hydrochloric acid. (15 cm 3 ). The organic phase was collected and dried over anhydrous magnesium sulphate. After evaporating the solvent, the residue was purified by column chromatography on a silica gel (eluting with dichloromethane/ethyl acetate=20:1) to give 2 (4.94 g, 24.5 mmol, 61% yield) as a crystalline white solid [45] : 1 H NMR (CDCl 3 ) δ 10.02 (s, 1H), 8.16 (d, 1H, J =8.4 Hz), 7.95 (dd, 1H, J =7.6 Hz), 7.80 (d, 1H, J =7.2 Hz), 6.05 (s, 1H), 2.75 (s, 3H), 2.31 (s, 3H). Anal. (calc.) for C 11 H 11 N 3 O ( 2 ): C, 65.43 (65.66); H, 5.61 (5.51); N, 20.56 (20.88)%. Preparation of 1,2-bis[6-(3,5-dimethyl-1H-pyrazol-1-yl)pyrid-2-yl]-2-hydroxy-ethanone (3) 2 (4.94 g, 24.5 mmol) was dissolved in ethanol (100 cm 3 ) and an aqueous solution (10 cm 3 ) of potassium cyanide (325 mg, 5.00 mmol) was added while the mixture was stirred. A yellow precipitate was collected by filtration and washed with a small amount of water and ethanol to give, after drying, the crystalline solid 3 (4.42 g, 11.3 mmol, 92% yield): 1 H NMR (CDCl 3 ) δ 12.01 (s, 2H), 7.95 (dd, 2H, J =8.0 Hz), 7.81 (d, 2H, J =7.8 Hz), 7.66 (d, 2H, J =8.0 Hz), 6.07 (s, 2H), 2.59 (s, 6H), 2.32 (s, 6H). 13 C NMR (100 MHz, CDCl 3 ) 154.09, 150.58, 149.94, 140.53, 139.77, 135.26, 117.42, 115.73, 109.27, 13.59, 13.53. Anal. (calc.) for C 22 H 22 N 6 O 2 ( 3 ): C, 65.53 (65.66); H, 5.60 (5.51); N, 20.73 (20.88)%. ESI–MS m/z (obs./calc. )=403.3/403.2 for [ 3 +H] + (C 22 H 23 N 6 O 2 ). Preparation of bis-[6-(3,5-dimethyl-1H-pyrazol-1-yl)pyrid-2-yl]glyoxal (4) 3 (4.42 g, 11.3 mmol) was dissolved in concentrated nitric acid (10 cm 3 ). After the evolution of nitrogen dioxide gas had subsided, the solution was neutralized with a saturated aqueous solution of potassium hydroxide. A precipitate was collected by filtration and purified by column chromatography on silica gel (eluting with dichloromethane/ethyl acetate=20:1) to give 4 (2.68 g, 6.69 mmol, 59% yield) as a pale yellow green solid: 1 H NMR (CDCl 3 ) δ 8.20-8.18 (m, 2H), 8.00-7.99 (m, 4H), 5.86 (s, 2H), 2.22 (s, 6H), 2.11 (s, 6H). 13 C NMR (100 MHz, CDCl 3 ) 196.46, 153.09, 150.68, 149.35, 141.92, 139.42, 119.83, 118.32, 109.94, 14.37, 13.56. Anal. (calc.) for C 22 H 20 N 6 O 2 ( 4 ): C, 66.04 (65.99); H, 5.12 (5.03); N, 20.98 (20.99)%. ESI–MS m/z (obs./calc. )=401.3 / 401.2 for [ 4 +H] + (C 22 H 21 N 6 O 2 ). Preparation of 2-phenyl-4,5-bis[6-(3,5-dimethyl-1H-pyrazol-1-yl)pyrid-2-yl]-1H-imidazole ( HL ) 4 (2.68 g, 6.69 mmol), benzaldehyde (743 mg, 7.00 mmol) and ammonium acetate (1.85 g, 24.0 mmol) were dissolved in acetic acid (80 cm 3 ) and refluxed for sixteen hours before cold water was added and the mixture was neutralized by addition of saturated sodium hydroxide solution. The resulting precipitate was extracted into dichloromethane, and the organic phase was dried over anhydrous magnesium sulphate. The solvent was removed in vacuo , and the residue was purified by alumina column chromatography (activity stage I, eluting with dichloromethane then methanol) to give HL (1.65 g, 3.38 mmol, 51% yield) as a white solid: 1 H NMR (CDCl 3 ) δ 11.16 (s, 1H), 8.20 (d, 1H, J =7.6 Hz), 8.03 (d, 2H, J =7.2 Hz), 7.00 (d, 1H, J =7.6 Hz), 7.91 (dd, 1H, J =8.0 Hz), 7.78 (d, 1H, J =8.0 Hz), 7.61 (dd, 1H, J =7.6 Hz), 7.50 (d, 1H, J =7.6 Hz), 7.49 (dd, 2H, J =7.4 Hz), 7.42 (dd, 1H, J =7.4 Hz), 6.06 (s, 1H), 5.93 (s, 1H), 2.66 (s, 3H), 2.32, (s, 6H), 2.28 (s, 3H). 13 C NMR (100 MHz, CDCl 3 ) 152.29, 151.87, 149.87, 149.70, 147.17, 146.37, 141.35, 140.69, 139.71, 139.01, 138.48, 129.73, 129.43, 129.15, 128.92, 125.67, 120.30, 120.23, 114.52, 114.25, 109.03, 108.80, 14.32, 13.91, 13.63, 13.62. Anal. (calc.) for C 29 H 26 N 8 ( HL ): C, 71.31 (71.59); H, 5.60 (5.39); N, 22.59 (23.03)%. ESI–MS m/z ( obs./calc. )=487.2/487.2 for [HL+H] + (C 29 H 27 N 8 ). Preparation of [Fe II 4 (L) 4 ] complex HL (97.3 mg, 0.20 mmol) in acetonitrile (5.0 cm 3 ) was added to Fe(BF 4 ) 2 ·6H 2 O (67.5 mg, 0.20 mmol) in acetonitrile (5.0 cm 3 ). Diethyl ether was allowed to diffuse into the solution, resulting in the formation of orange blocks and yellow needle crystals. The crystals were then washed with methanol, and the yellow crystals removed. The orange crystals of [Fe II 4 ] (BF 4 ) 4 ·2CH 3 CN were collected by filtration (31.5 mg, 0.013 mmol, 25% yield). Anal. (calc.) for C 116 H 100 N 32 B 4 F 16 Fe 4 ( [Fe II 4 ] (BF 4 ) 4 ): C, 55.32 (55.44); H, 4.31 (4.01); N, 17.70 (17.84)%. ESI–MS m/z (obs./calc. )=541.5/541.4 for [ M –4(BF 4 )] 4+ (C 116 H 100 N 32 Fe 4 ). The 57 Fe-enriched samples for Mössbauer spectra measurements ware prepared using metallic 57 Fe foils (95.5%). Preparation of [Fe III 2 Fe II 2 (L) 4 ] complex Excess AgBF 4 (12.0 mg, 0.062 mmol) was added to a nitromethane (5.0 cm 3 ) solution of [Fe II 4 ] (31.5 mg, 0.013 mmol). The mixture was stirred for 15 min at 50 °C, cooled to room temperature, and the precipitate (silver) removed by filtration. Diethyl ether was allowed to diffuse into the filtrate, resulting in the formation of dark red rhombic crystals of [Fe III 2 Fe II 2 ](BF 4 ) 6 ·6CH 3 NO 2 ·(C 2 H 5 ) 2 O·4H 2 O, which were collected by filtration (28.1 mg, 0.009 mmol, 74% yield). Anal. (calc.) for C 123 H 127 N 35 B 6 F 24 Fe 4 O 11 ([Fe III 2 Fe II 2 ](BF 4 ) 6 ·3CH 3 NO 2 ·(C 2 H 5 ) 2 O·4H 2 O): C, 49.25 (48.99); H, 4.18 (4.24); N, 15.97 (16.26)%. Details of magnetic measurements on [Fe II 4 ] The χ m T value of [Fe II 4 ] at 100 K (↑) was 6.89 e.m.u. mol −1 K, close to the spin-only value of 6.63 e.m.u. mol −1 K ( g =2.10), calculated from the sum of the uncorrelated spins of two HS-Fe II ( S =2) and two LS-Fe II ( S =0) ions, as predicted by the structural and Mössbauer data. As the sample was heated, the χ m T value rapidly increased. At 190 K (↑), the χ m T plot showed a small step with a value of 10.57 e.m.u. mol −1 K, closely corresponding to the spin-only value of 9.95 e.m.u. mol −1 K expected for an average of three HS-Fe II ions and one diamagnetic LS-Fe II centres per molecule. On further heating to 300 K, the magnetic susceptibility reached a plateau with a χ m T value of 13.26 e.m.u. mol −1 K, suggesting that all iron ions were in their HS states above 250 K. Subsequent measurements in cooling mode echoed the two-step heating profile, but with a relatively wide thermal hysteresis. Mössbauer measurements ( Supplementary Fig. 3 ) and structural analyses confirmed that the decrease in χ m T values below 100 K was not due to SCO behaviour, but more likely a consequence of the antiferromagnetic interactions between the HS iron ions. The thermal hysteresis and multi-step phase transition mean that [Fe II 4 ] is a thermally multi-bistable molecule with the spin-state conversions of [(LS-Fe II ) 2 (HS-Fe II ) 2 ] ⇄ [(LS-Fe II )(HS-Fe II ) 3 ] ⇄ [(HS-Fe II ) 4 ]. Accession codes The X-ray crystallographic coordinates for structures reported in this Article have been deposited at the Cambridge Crystallographic Data Centre (CCDC), under deposition numbers CCDC 980494-980501. These data can be obtained free of charge from The Cambridge Crystallographic Data Centre via www.ccdc.cam.ac.uk/data_request/cif . How to cite this article: Matsumoto, T. et al. Programmable spin-state switching in a mixed-valence spin-crossover iron grid. Nat. Commun. 5:3865 doi: 10.1038/ncomms4865 (2014).